Stabilizing colloidal crystals by leveraging void distributions Colloids often crystallize into polymorphic structures, which are only separated by marginal differences in free energy. Due to this fact, the face-centred cubic and hexagonal close-packed hard-sphere morphologies, for example, usually crystallize simultaneously from a supersaturated solution. The resulting lack of long-range order in these polymorphic structures has been a significant barrier to the widespread application of these crystals in, for instance, photonic bandgap materials. Here, we report a simple method to stabilize one out of two competing polymorphs by exploiting the fact that they have significantly different spatial distributions of voids. We use a variety of polymeric additives whose geometries can be tuned such that their entropy loss, which is related to crystal void symmetries, is different in the two competing polymorphs. This, in turn, controls which polymorph is most thermodynamically stable, providing a generalizable means to stabilize a selected crystal polymorph from a suite of competing structures. Colloidal crystals with well-defined global order have utility in a range of novel optical and catalytic devices [1] , [2] , [3] , for example, as photonic bandgap materials. However, such long-range order is often difficult to achieve in practice since the structure of these crystals, determined by short-range interactions, is generally polymorphic. For instance, in the limiting case of hard spheres, crystals are known to form hybrids of hexagonal close-packed (HCP) and face-centred cubic (FCC) structures [4] , [5] , [6] , [7] , [8] . This is due to the fact that the FCC structure is only ~0.001 k B T per sphere higher in entropy [9] , [10] , [11] . While the energy, pressure and overall packing fraction of the FCC and HCP structures are the same as a consequence of having an identical number of nearest neighbors, the manner in which their voids distribute the free volume inside each crystal is not ( cf . Fig. 1 ). 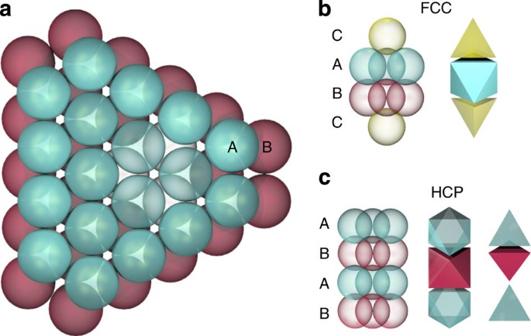Figure 1: Crystal morphologies. (a) Two adjacent layers, A and B, of the FCC and HCP crystals are identical. The eclipsed HCP configuration repeats this stacking pattern and has ABAB symmetry, while rotating a third plane by 60° yields the staggered FCC polymorph (ABC symmetry). Stacking faults (for example, ABCBA) create ‘random’ hexagonal close-packed structures (rHCP). The interstitial voids between neighbouring planes can be described by two types of platonic solids: octahedrons and tetrahedrons. (b) The voids in these crystals are connected out-of-plane in very different manners: in the FCC structure, octahedral voids (OVs) do not share any common faces and any direct connection between neighbouring OVs is interrupted by intervening tetrahedral voids (TVs), (c) whereas in the HCP crystal OVs do share common faces, providing a direct route from one OV to another. Figure 1: Crystal morphologies. ( a ) Two adjacent layers, A and B, of the FCC and HCP crystals are identical. The eclipsed HCP configuration repeats this stacking pattern and has ABAB symmetry, while rotating a third plane by 60° yields the staggered FCC polymorph (ABC symmetry). Stacking faults (for example, ABCBA) create ‘random’ hexagonal close-packed structures (rHCP). The interstitial voids between neighbouring planes can be described by two types of platonic solids: octahedrons and tetrahedrons. ( b ) The voids in these crystals are connected out-of-plane in very different manners: in the FCC structure, octahedral voids (OVs) do not share any common faces and any direct connection between neighbouring OVs is interrupted by intervening tetrahedral voids (TVs), ( c ) whereas in the HCP crystal OVs do share common faces, providing a direct route from one OV to another. Full size image Polymers are commonly used as depletants in colloidal systems, and binary colloid–polymer mixtures have been exhaustively studied for the past half century [12] , [13] , [14] , [15] , [16] , [17] , [18] , [19] , [20] . The phenomenon of depletion is a manifestation of size-asymmetric, athermal, binary systems maximizing their entropy; the volume ‘freed’ when the larger species aggregates produces a disproportionate increase in the entropy of the smaller species (depletant) compared to the entropy lost by the larger species [21] , [22] . At high-enough polymer densities this is sufficient to drive phase separation, in which both the colloids and polymers partition into complementary rich and lean phases. In this work, the colloid-rich (polymer-lean) phase we focus on is the crystal phase, which is in equilibrium with a dense polymer phase containing dilute colloids (colloidal ‘gas’) [14] . In previous studies, the nature of the polymers adsorbed in the voids of the colloidal crystal has been neglected on the assumption that the polymers’ contribution to the system’s free energy is inconsequential [14] , [19] , [23] . However, when a depletant is confined into such restricted environments as the interstices of a crystal, its topology implies that it can have very different entropies in the different polymorphs (which have different spatial void distributions). This effect is driven by local asymmetries at the length scale of the next-nearest neighbour stacking plane in the crystal (AB X , where X can be either A or C), and thus is entirely overlooked by mean-field theories. Here we show that such differences in void symmetry play a significantly underappreciated role in determining the free energy of depletants adsorbed in the crystal, which can be exploited to bias the production of a single polymorph over others during crystallization. Because the specific free energies of pure FCC and HCP crystals differ only marginally, we find that these differences in chain entropy provide a sufficient driving force to uniquely select a single polymorph. Our equilibrium methodology promises to obviate other exotic techniques, such as templating [1] , gravity reduction [8] , [24] , anisotropic thermal interactions [25] , [26] or thermal gradients [27] , for selecting a desired crystal structure from a suite of competitors. This constitutes a novel, but simple design principle whereby a depletant’s geometry may be tailored to select a specific polymorph without any modification of the colloid itself; we illustrate this principle with two examples: (1) for linear polymers as depletants, and (2) for size-asymmetric block copolymers. Going further, we propose that our logic is generalizable to other depletant topologies as well. Polymorph discrimination with linear homopolymers First, we consider mixtures of hard-sphere colloids and linear polymers. In the absence of polymer, or for very short chains, hard spheres are experimentally observed to always crystallize into the random hexagonal close-packed (rHCP) structure [4] , [28] , though computer simulations suggest they may anneal to the more stable FCC polymorph over much longer timescales [7] . In contrast, for polymers long enough to span two (or more) neighbouring crystal voids our simulations show that the HCP crystal is strongly stabilized relative to the FCC, and becomes overwhelmingly the most thermodynamically (and kinetically) favoured state. To understand why, we first consider the free energy difference between polymers adsorbed in each type of crystal. In our model system, polymers are treated as fully flexible bead-spring necklaces of M beads, each of diameter σ m =1, while colloids are represented as large spheres of diameter σ c =6.45, unless otherwise stated. All spheres interact with a purely repulsive Weeks-Chandler-Andersen (WCA) potential (which is a Lennard–Jones potential truncated at its minimum and shifted, cf . Methods, Model A). By performing Monte Carlo (MC) simulations to insert a single polymer segment-by-segment into these crystals we measured the excess incremental chemical potential, , of an adsorbed chain [29] . The sum of the incremental chemical potentials provides the total excess chemical potential of the chain, , which is a measure of the accessible volume inside each crystal ( Fig. 2 ). For M =1, a successful insertion depends on locating voids in the crystal that only represent roughly 26% of the volume of the simulation cell. However, subsequent insertions benefit from the fact that the first bead has already been successfully inserted into a void. Thus, these beads have a disproportionately larger free volume in their immediate vicinity, and are therefore incrementally easier to insert than the first. As the local void fills up, the chain has to find another void to occupy. Once this happens, for the FCC crystal begins to exceed that of the HCP, in this case for M ≥10. We focus on M =10 because it is the shortest chain that produces a statistically significant difference between the polymorphs. Though small, this difference (roughly 0.1 k B T in favour of the HCP) is two orders of magnitude larger than the entropy difference in favour of the FCC state based on the pure colloid case [9] , [10] , [11] . The origin of this result lies in the differences between the crystal void symmetries. 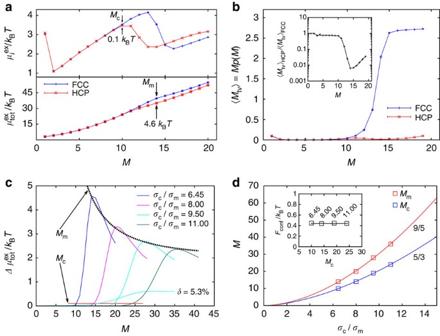Figure 2: Thermodynamics of a confined linear homopolymer. (a) Incremental,, and total,, excess chemical potential of a polymer of lengthMinside rigid crystals (cf. Methods). ForM<10, the chemical potentials of chains in each polymorph are identical within statistical error (95% confidence), while forM>10, their difference rises to the order of unity or more in favour of the HCP crystal. ForM=Mc=10 the difference is roughly 0.1kBT.Mmdenotes the chain length when the difference inbetween the polymorphs is at a maximum. (b) The average number of monomers found in tetrahedral voids (TVs) in each polymorph (the remainder are in octahedral ones) when the chain has a total length,M.p(M) is the normalized probability for each monomer that resides in a TV when the chain is of lengthM. The inset shows the ratio between the polymorphs; clearly, in the HCP crystal the monomers are almost two orders of magnitude less likely to occupy the highly confining TVs and instead expand into neighbouring OVs whenMis sufficiently large. (c) A plot of the difference in total excess chemical potential between the two polymorphs,, as a function of total polymer chain length at four different ratios ofσc/σm. The red line indicates the location ofMc(where the difference exceeds 0.1kBT) and the dashed black line is a fit ofMmto the form, implying a limiting value of. The dashed cyan line indicates results forσc/σm=9.50 with a polydispersityδ=5.3% (cf. Methods). (d)McandMmversus the ratio of the colloid and monomer diameters. Each follows a (different) scaling law as the colloid–monomer size asymmetry grows, suggesting that the effect will still be present as the colloid becomes much larger than a monomer (Kuhn) segment. The inset depicts the free energy according to equation (1) versusMcat four differentσc/σmratios; its constant value validates the scaling equation and implicates confinement effects as the cause of the differences inbetween the polymorphs. Figure 2: Thermodynamics of a confined linear homopolymer. ( a ) Incremental, , and total, , excess chemical potential of a polymer of length M inside rigid crystals ( cf . Methods). For M <10, the chemical potentials of chains in each polymorph are identical within statistical error (95% confidence), while for M >10, their difference rises to the order of unity or more in favour of the HCP crystal. For M = M c =10 the difference is roughly 0.1 k B T . M m denotes the chain length when the difference in between the polymorphs is at a maximum. ( b ) The average number of monomers found in tetrahedral voids (TVs) in each polymorph (the remainder are in octahedral ones) when the chain has a total length, M . p ( M ) is the normalized probability for each monomer that resides in a TV when the chain is of length M . The inset shows the ratio between the polymorphs; clearly, in the HCP crystal the monomers are almost two orders of magnitude less likely to occupy the highly confining TVs and instead expand into neighbouring OVs when M is sufficiently large. ( c ) A plot of the difference in total excess chemical potential between the two polymorphs, , as a function of total polymer chain length at four different ratios of σ c / σ m . The red line indicates the location of M c (where the difference exceeds 0.1 k B T ) and the dashed black line is a fit of M m to the form , implying a limiting value of . The dashed cyan line indicates results for σ c / σ m =9.50 with a polydispersity δ =5.3% ( cf . Methods). ( d ) M c and M m versus the ratio of the colloid and monomer diameters. Each follows a (different) scaling law as the colloid–monomer size asymmetry grows, suggesting that the effect will still be present as the colloid becomes much larger than a monomer (Kuhn) segment. The inset depicts the free energy according to equation (1) versus M c at four different σ c / σ m ratios; its constant value validates the scaling equation and implicates confinement effects as the cause of the differences in between the polymorphs. Full size image While both the FCC and HCP crystals have two tetrahedral (TV) and one octahedral void (OV) per colloid, their relative arrangements are very different ( cf . Fig. 1 ). In both FCC and HCP crystals, in the plane of the hexagonally ordered colloids, the voids that share faces follow the connectivity pattern: OV–TV–OV–TV. On the other hand, in the out-of-plane direction in the HCP crystal, the OVs stack on top of themselves as do the TVs. Therefore, in the HCP crystal a chain can ‘travel’ normal to the hexagonally packed planes directly from one OV to another since they share common faces. In contrast, the staggered configurations of the A and C planes in the FCC crystal imply that each OV face is ‘capped’ by TVs in all directions, and thus there are no direct OV–OV pathways. The significance of this void connectivity difference is appreciated by calculating the total volume of each void. As an approximation, consider the largest sphere, of radius r , that could be inscribed into each type of void without overlapping the colloids that form the vertices. If the length of each edge is σ c , then for TVs , while for OVs . Therefore OVs have over (0.414/0.225) 3 ≳ 6 times the volume of their TV counterparts. Sufficiently long chains cannot exist in a single void and must cross the faces of the void polyhedra through trigonal gaps formed by triplets of colloids in order to find more room; at the size asymmetry of the model system ( σ m / σ c ≈0.155) each gap is just wide enough to allow a single bead through at a time. The chain thus incurs a significant entropic penalty every time it must do so. In the HCP crystal only, vertical OV stacking symmetry permits a chain to move directly from one OV to another allowing chains that require multiple voids ( M ≥10) to access significantly more volume with lower entropic penalties than in the FCC state. This picture suggests the point at which the polymer begins to explore, if not completely cross over to, a neighbouring OV in the HCP polymorph is where μ tot ex becomes sufficiently disparate between the two crystals. In fact, by explicitly measuring the average number of monomers found in TVs as the chain grows, 〈 M tv 〉, we have confirmed this hypothesis. Consider Fig. 2b ; for both polymorphs, as the chain exceeds a length of 2, the TVs become significantly more confining than the available OVs, which the chain almost exclusively occupies until it reaches M =10. Surrounded by only TVs, polymers in the FCC crystal do not cross between voids until M ≈13, and do not reach the next OV until M ≈15. However, the HCP polymorph provides a large, easily accessible amount of free volume in the neighbouring OV voids, and does not require a growing chain to traverse any TVs; only as a single OV fills up do chain ends appear to occasionally sample the TV space, and once the chain finds the next OV it rarely returns to visit its neighbouring TVs. Clearly this effect is quantitatively dependent upon the mutually excluded volume between the monomers (Kuhn segments) and colloids. However, upon varying the colloid to monomer diameter ratio, we found that this effect did not disappear as the asymmetry increased. The magnitude of the maximum difference between the two polymorphs tends to both decay and occur at larger M , but plateaus to a limiting value of roughly 2 k B T ( cf . Fig. 2 ). This suggests that as σ c / σ m increases the picture will not qualitatively change ( cf . Supplementary Fig. 1 ), and that there will always exist a critical length, M c , beyond which a chain will be able to sense the different local environments inside each polymorph. If we take M c to be the point at which the difference in between the two polymorphs is roughly 0.1 k B T , we find that these chain lengths follow macroscopic scaling laws for confined polymers. Namely, the free energy of confinement, F conf / k B T , for an athermal polymer should scale as ( cf . Supplementary Note 1 for derivation): The right-hand side of equation (1) is plotted in the inset of Fig. 2d . As expected, this quantity is constant across all size asymmetries; this equation may also be interpreted as a statement of how large the polymer must be to perforate an OV, since for a single chain in a good solvent R g ~ M 3/5 σ m . This supports the conclusion that the difference in polymer free energy between the two polymorphs is driven by confinement in different local environments. Further, once a chain is sufficiently long such that the free energy to confine it in an OV exceeds a fixed threshold, the chain will bias the system toward the HCP polymorph. Therefore, as σ c / σ m increases to more experimentally realizable scales, we do not expect this effect to disappear. Furthermore, the chain length, M m , where the weak maximum in the difference of between the polymorphs ( Fig. 2d ) is observed, also scales as a power law: Phase behaviour and crystal grain structure These results suggest that for this model when M ≥10 a depletion-flocculated colloidal crystal will thermodynamically favour the HCP crystal over the FCC. To confirm this prediction, we studied the crystal–vapour equilibrium of nearly hard-sphere colloids with monodisperse polymers of chain length, M =10 ( q =2 R g / σ c ≈0.5), using canonical molecular dynamics (MD) simulations. Initially amorphous mixtures were used and we observed a clear structural transition between amorphous and crystalline states. 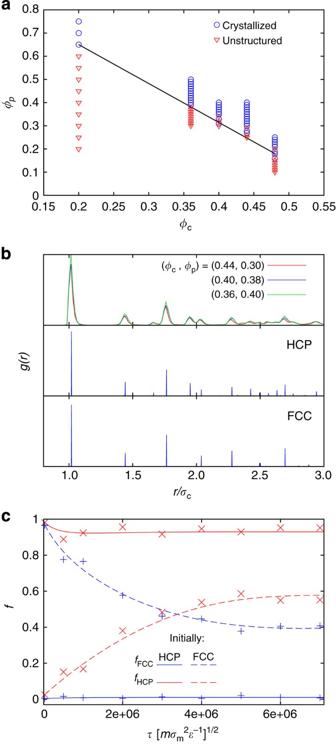Figure 3: Phase behaviour and structure of crystallizing colloids. (a) Phase diagram in the colloid volume fraction–polymer volume fraction (ϕc−ϕp) plane forσc/σm=6.45 (cf. Methods, Model A), whereM=10. We defineand, whereRgis the polymer’s infinitely dilute radius of gyration andρpandρcare the polymer and colloid number densities, respectively. The black line is a guide to the eye. (b) Radial distribution functions,g(r), for crystallized colloids at three state points. Perfect FCC and HCP states are shown in the bottom panels, while the top panel depicts measured behaviour whenM=10. Only the colloids classified as crystallized (cf. Methods) are included. (c) Fraction,f, of the colloids present as each polymorph as determined by bond order parameter analysis. Approximately spherical FCC and HCP crystallites at an overall volume fraction ofϕc=0.2 were placed in solution withM=10 polymers atϕp=0.65. The initially FCC state gradually evolved towards the HCP state, while HCP crystals remained unchanged over the same time, illustrating that the HCP is truly the most stable state. Figure 3a is in reasonable agreement with both theory [19] and experiments [23] for similar q , for crystal–vapour and liquid–vapour phase boundaries in the plane of polymer and colloid volume fractions, ϕ c − ϕ p . A caveat is that these results are subject to the relatively slow nucleation kinetics near the binodal [28] . Figure 3: Phase behaviour and structure of crystallizing colloids. ( a ) Phase diagram in the colloid volume fraction–polymer volume fraction ( ϕ c − ϕ p ) plane for σ c / σ m =6.45 ( cf . Methods, Model A), where M =10. We define and , where R g is the polymer’s infinitely dilute radius of gyration and ρ p and ρ c are the polymer and colloid number densities, respectively. The black line is a guide to the eye. ( b ) Radial distribution functions, g ( r ), for crystallized colloids at three state points. Perfect FCC and HCP states are shown in the bottom panels, while the top panel depicts measured behaviour when M =10. Only the colloids classified as crystallized ( cf . Methods) are included. ( c ) Fraction, f , of the colloids present as each polymorph as determined by bond order parameter analysis. Approximately spherical FCC and HCP crystallites at an overall volume fraction of ϕ c =0.2 were placed in solution with M =10 polymers at ϕ p =0.65. The initially FCC state gradually evolved towards the HCP state, while HCP crystals remained unchanged over the same time, illustrating that the HCP is truly the most stable state. Full size image The resulting configurations were analysed using Steinhardt–Nelson bond order parameters to characterize crystal grains based on their local orientational symmetry ( cf . Methods) [30] , [31] . After sufficient time, the radial distribution function between crystallized colloids was identical for all system densities above the line given in the phase diagram ( Fig. 3a ), indicating a unique final state. A representative configuration is depicted in Supplementary Fig. 2 . However, this state is clearly not the FCC crystal as assumed by mean-field theories; instead, it is apparent from the location and relative size of the peaks in Fig. 3b that the resulting structure is HCP. For pure colloids, the Ostwald ‘rule of stages’ posits that crystallization from a supernatant solution should proceed via a series of metastable intermediate states [16] , namely, a progression from a body-centred cubic (BCC) crystal to HCP and finally a very slow transition to pure FCC, during which the crystal appears to have rHCP character [4] , [8] , [31] , [32] . Although recent studies have challenged the ability of this principle to predict the outcome of specific nucleation events, the importance of metastable intermediates has been verified even for soft colloids [33] , [34] , [35] . Thus, one could hypothesize that the HCP state observed here might simply be metastable. To dispel this notion, we repeated simulations at the same overall colloid and polymer densities, but initialized the colloids as either perfect FCC or HCP crystals. Using bond order parameter analysis we classified each colloid in the simulation as FCC, HCP, liquid, or unknown ( cf . Methods). Initially, some amount of polymer, depending on the ϕ p (external osmotic pressure), invades each crystal ( cf . Supplementary Note 2 and Supplementary Fig. 3 ); as polymers explore the free volume inside the crystal, they begin to recognize the entropic favourability of the HCP configuration over the FCC, which would suggest a slow transition from the FCC to the HCP polymorph. As Fig. 3c illustrates, the initially FCC crystals do, in fact, reorder into the HCP state, while the initially HCP crystals remain stable over the same amount of simulation time. Generalization to arbitrary depletant topology We have also found that this effect can be generalized to other depletant topologies. For instance, although the HCP polymorph is always predicted to be the most stable when using linear polymer chains (of sufficient length) as depletants, one can imagine other topologies that may favour the FCC. We focus here on the case of asymmetric tetramers, that is, a four-bead chain whose inner two monomers have a diameter of unity ( σ m =1.0), but whose terminal beads have a diameter of 1.75 σ m ( cf . Methods, Model B and Fig. 4 ). The bond lengths between the end and middle beads are indicated as r end and r mid , respectively. To a first approximation this represents a block copolymer whose different constituents are experiencing good and poor solvent interactions. 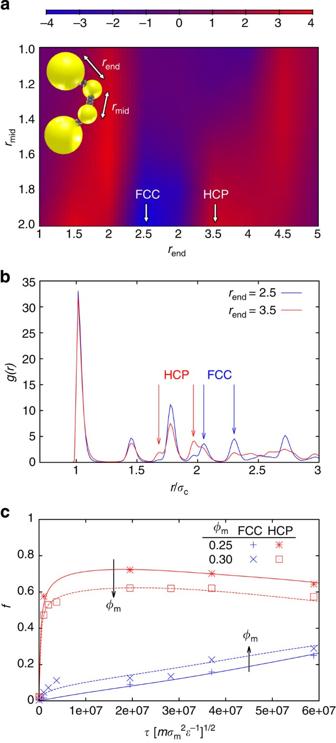Figure 4: Depletion driven by asymmetric tetramers. (a) Difference in the total excess chemical potential of the fully inserted tetramer between the close-packed polymorphs., so that red (positive) indicates a preference for the HCP, while blue (negative) indicates a preference for the FCC. Hereσc/σm=6.45. A tetramer is shown schematically to illustrate the basic geometry; large beads at the end have a diameter of 1.75σm, while the two inner beads each have a diameter ofσm=1.0 (cf. Methods, Model B). (b) The radial distribution function for all colloids present in each system at the end of the MD simulations (5e7τ) corresponding to (a) whenϕc=0.2 and the monomer volume fraction,ϕm=4πρt(2(σm/2)3+2(1.75σm/2)3)/3 =0.15, whereρtis the number density of the tetramers. HCP peaks are present in the case ofrend=3.5, but are suppressed in the case ofrend=2.5, where the FCC peaks emerge. (c) Fraction of colloids present as each type of polymorph according to bond order parameter analysis in a MD simulation of tetramers using Model C (cf. Methods). The beads on the ends are slightly larger (2.2σm) and bonds a bit shorter, which seems to relax some of the kinetic barriers to crystallization. Both samples clearly anneal to the FCC state in an approximately linear fashion, and larger tetramer densities tend to both reduce the amount of HCP polymorph which initially nucleates, and facilitate the annealing process. Hereϕc=0.2 andϕm=4πρt(2(σm/2)3+2(2.2σm/2)3)/3. Figure 4: Depletion driven by asymmetric tetramers. ( a ) Difference in the total excess chemical potential of the fully inserted tetramer between the close-packed polymorphs. , so that red (positive) indicates a preference for the HCP, while blue (negative) indicates a preference for the FCC. Here σ c / σ m =6.45. A tetramer is shown schematically to illustrate the basic geometry; large beads at the end have a diameter of 1.75 σ m , while the two inner beads each have a diameter of σ m =1.0 ( cf . Methods, Model B). ( b ) The radial distribution function for all colloids present in each system at the end of the MD simulations (5e7 τ ) corresponding to ( a ) when ϕ c =0.2 and the monomer volume fraction, ϕ m =4 πρ t (2( σ m /2) 3 +2(1.75 σ m /2) 3 )/3 =0.15, where ρ t is the number density of the tetramers. HCP peaks are present in the case of r end =3.5, but are suppressed in the case of r end =2.5, where the FCC peaks emerge. ( c ) Fraction of colloids present as each type of polymorph according to bond order parameter analysis in a MD simulation of tetramers using Model C ( cf . Methods). The beads on the ends are slightly larger (2.2 σ m ) and bonds a bit shorter , which seems to relax some of the kinetic barriers to crystallization. Both samples clearly anneal to the FCC state in an approximately linear fashion, and larger tetramer densities tend to both reduce the amount of HCP polymorph which initially nucleates, and facilitate the annealing process. Here ϕ c =0.2 and ϕ m =4 πρ t (2( σ m /2) 3 +2(2.2 σ m /2) 3 )/3. Full size image Although the design space is vast, we found that the two bond lengths were sufficient to control which polymorph is most stable. We repeated the incremental chemical potential MC analysis with varying bond lengths to produce the plane shown in Fig. 4a . This illustrates the difference in the total excess chemical potential of the tetramers when fully inserted into each of the two polymorphs, and suggests that at ( r mid , r end )=(2, 2.5) the FCC polymorph should be strongly favoured while at (2, 3.5) the HCP should be favoured instead. Again we tested these predictions with canonical MD simulations, as shown in Fig. 4b , which clearly confirmed these conjectures. As the terminal monomers of a tetramer are too large to fit through the trigonal gaps formed by tangent colloids in either of the close-packed morphologies, the precipitation of the colloids proceeds via a ‘co-crystallization’ route whereby the colloids crystallize around the tetramers. This leads to slower dynamics, which are more sensitive to nucleation events than in the case of linear chains, but nonetheless behave as expected. We tested the predictive capacity of this method for other tetramers as well and found, in all cases, the MC method to be a robust predictor of the most stable polymorph. By increasing the diameter of the terminal beads and shortening the bonds (Model C) we found that kinetic barriers tended to be reduced. Figure 4c illustrates this for conditions where (FCC preference). To our knowledge, there has not been a clear experimental realization of this phenomenon for several reasons. External factors such as difficulty in simultaneous density matching of both colloids and depletants [28] and thermal interactions between monomer (Kuhn) segments and the colloids are likely to play an important role. The former is known to affect the kinetics of crystallization in terrestrial environments [8] , [28] , while the latter can disrupt this effect if the cross-interactions are significant enough; however, the present work illustrates that entropy alone is sufficient to provide a mechanism that can discriminate between polymorphs. We further considered the effects of colloidal polydispersity on this phenomenon ( cf . Methods). Although this effect has been shown to not affect the relative stability of the FCC and HCP polymorphs in pure systems [36] , it is conceivable that the resulting void distortions in the polydisperse crystals could significantly impact our results. As a first approximation, we repeated our MC simulations for σ c / σ m =9.50 with a bidisperse population of colloids, where half had a diameter of 9.50 σ m while the diameter of the other half (chosen at random) was reduced by 10%. This leads to a polydispersity of δ =5.3%, which is commensurate with the largest polydispersity observed in hard-sphere crystals [37] , [38] . Although simulations suggest that hard-sphere fluids of arbitrary polydispersity can be coaxed into precipitating crystalline solids at sufficiently high pressures, fractionation tends to prevent the crystals from exceeding a polydispersity of roughly 6% [38] , [39] . In our simulations, we leave the colloids placed at the original lattice positions they would be found at if the system were monodisperse with σ c / σ m =9.50, which opens the crystal significantly. In a real crystal, we would expect the lattice to deform and compress, making the polymer confinement even more dramatic. Of course, we expect this effect to be identical in both polymorphs, so we interpret our results as an upper bound for the impact of colloidal polydispersity on negating our results. Figure 2c clearly illustrates that the magnitude of the difference in polymer chemical potential between the two polymorphs remains on the order of k B T , and thus colloidal polydispersity does not destroy this phenomenon. Remarkably, although polydispersity may weaken the overall magnitude of the effect at M m , we note that M c slightly decreases, suggesting that in polydisperse systems this distinction between the polymorphs may occur at even shorter chain lengths than in more monodisperse ones. Our work provides useful guidelines for identifying an experimentally realizable system exhibiting this phenomenon. Our results show that this effect is the most noticeable when σ c / σ m is small. Thus, polymers with large Kuhn segments in combination with small colloids are the most promising means of observing the phenomena discussed here; for example, our results for σ c / σ m =9.50 in Fig. 2c would be analogous to a system of double-stranded DNA and colloids with a diameter of ~1 μm. Differentiation between crystal polymorphs via the interplay of depletants and void symmetry has many important potential applications, especially in self-assembling photonic nanostructures where long-range crystalline order is crucial. Inducing spontaneous long-range order in colloidal crystals traditionally requires the assistance of exotic external mechanisms [1] , [8] , [24] , [25] , [26] , [27] . However, our results illustrate that intrinsic differences in spatial void distributions can be exploited by a polymer, or other well-designed depletants confined in the crystal phase, to thermodynamically select a morphology without the need for such intensive techniques. The use of confined depletants to mediate colloidal crystal structure may thus provide a generally applicable design mechanism for the self-assembly of globally ordered crystal lattices. Bond order parameter analysis In a simulation, colloids are classified as solid, liquid or gas-like based on bond-orientation order parameters [30] , [31] . For systems that were observed to crystallize in Fig. 3 (Model A), we analysed the radial distribution function of the colloids to locate the first minimum immediately following the nearest-neighbour peak. This was generally constant at approximately r n =7.65, but was observed to vary by as much as ±0.5 with system density. Colloids within r n of each other are considered neighbours. The vector connecting any two neighbours, r ij , is considered a ‘bond’ whose orientation is characterized by the unit vector , which defines both a polar and azimuthal angle, θ ij and ϕ ij , respectively. This defines the l th degree spherical harmonic of order m , . The local structure around the i th colloid with N b ( i ) neighbors can be described by Following ref. 31 we focus on l =6 to quantify the degree of local ordering requisite of a solid rather than a liquid, which also exhibits non-zero local order. A normalized complex vector for each colloid, q 6 ( i ), can thus be defined with (2 × 6+1) orthogonal components: A dot product can then also be constructed as where the asterisk superscript denotes the complex conjugate [31] . If the dot product exceeds a given threshold, we define the two colloids as ‘connected’, and if a colloid has enough connections we consider it to be a solid particle. We took thresholds for the dot product and number of connections, q thresh and N n , to be 0.55 and 4, respectively. These values yielded unambiguous radial distribution functions characteristic of each phase ( cf . Supplementary Fig. 4 ), and are consistent with previously employed values for similar applications [6] , [31] , though further investigation revealed that the qualitative results of our analysis are somewhat insensitive to the absolute value of these parameters. A similar procedure can be used to identify the specific polymorph a crystallized colloid is present in. As described in ref. 40 , performing a simple averaging of the local bond order parameters for each colloid over its nearest neighbours tends to separate the regions of this phase space where the FCC and HCP (and other simple) crystal structures reside. The locally averaged bond order parameters are defined as where The quantity refers to the number of nearest neighbours around a colloid, i , including itself. Pure FCC, HCP, BCC and liquid structures were analysed with this technique to produce a unique ‘fingerprint’ in the plane for each, which was later used to classify our colloids during a simulation ( cf . Supplementary Fig. 5 and Supplementary Note 3 ). An analysis of the colloids’ radial distribution function qualitatively verified our results as well ( cf . Supplementary Fig. 6 and Supplementary Note 4 ). Monte Carlo Incremental excess chemical potential calculations for the polymers were performed by growing a chain, bead-by-bead, inside each type of crystal using MC techniques as described in ref. 29 . These crystals were initialized such that nearest neighbours were separated by σ c + g = σ c +2 1/6 −1 (cutoff of equation (8)), which was confirmed with subsequent MD simulations to be the equilibrium separation between nearest neighbours in the crystal. This creates a gap, g ≈0.12, beyond the hard-sphere diameter between nearest neighbours. We investigated this in more detail, but found that changing this gap size to span a typical range found in MD simulations did not change our results qualitatively ( cf . Supplementary Fig. 7 and Supplementary Note 5 ). All simulations were performed at a reduced temperature, T *= k B T / ε =1. Pair potentials are reported in the following subsections for each model we employed. Each polymer was grown inside a repeatable unit of each polymorph. The FCC environment was composed of 32 colloids arranged into stacked planes with ABC symmetry ( cf. Fig. 1 ) in a cubic, periodic box of length, . The HCP polymorph required a periodic, rectangular box of dimensions , in order to place four layers in ABAB symmetry for a total of 64 colloids. MC cycles of 5 × 10 6 −50 × 10 6 equilibration moves were performed per monomer currently in the system before a new monomer was formally grown on the chain. During each cycle the excess chemical potential measurements were performed by inserting a new ‘ghost’ monomer after roughly each of 1 × 10 4 successful relaxation moves. We employed simple monomer displacements, displacements of the polymer’s centre of mass and cut-and-regrowth schemes using Rosenbluth sampling accepted according to the Metropolis criterion [41] . The first move type was found to be sufficient to sample by brute force, though the latter two routines were helpful in refining the sampling of the probability that monomers occupied a TV when the chains became very long. This probability was measured during the equilibration period as was being calculated, but only the ensemble of beads that were fully inserted (no ghost beads) contributed to this measurement. Molecular dynamics Canonical (NVT) MD simulations to observe colloidal crystallization induced by linear polymers in Fig. 3a were run for more than 200 million time steps of length , and were initialized from low-density states equilibrated with Brownian dynamics, then quickly compressed to reach a final cubic box with sides of length L =50 σ m . All simulations were performed at a reduced temperature, T *= k B T / ε =1.0, using a Nosé–Hoover thermostat with a coupling constant of τ Q =1.0. The same thermostat, timestep and box size were used for all other MD simulations as well, such as those involved in melting a certain polymorph and to study crystallizing tetramers. This typically provided several hundred colloids, and several thousand polymers in each simulation. Crystallization was usually observed within the first quarter of the total simulation window for those used in Fig. 3a , but simulations were continued to verify the stability of the observed state. Of course, we suspect that crystallization can still be observed at lower ϕ p than what we report in Fig. 3a simply due to kinetic effects and the finite length of our simulations, which excludes nucleation events that could take a very long time to observe. Due to the low interfacial tension between the phases, we were unable to identify any fluid–fluid phase separation at lower densities within a reasonable time frame. Fluid–fluid phase separation at q =2 R g /σ c =0.5 is known to exist; however, a description of these phases is beyond the scope of this work. To reach effective timescales sufficient to observe crystallization, the mass of both the polymer beads and colloids, m , was set to unity, and all simulations were accelerated on graphics processing units with the open-source Highly Optimized Object-oriented Many-particle Dynamics package [42] , [43] . Even so, simulations at the level of full monomeric detail of the polymer required an extremely long time to generate the trajectories presented here. For instance, the melting simulations presented in Fig. 3c took over 30 days of wallclock time, while those in Fig. 4b took nearly 2 months; this simply serves to highlight the importance of our MC simulations, which required only a fraction of this time to search through a much broader parameter space. Polydispersity We emulated the effect of colloidal polydispersity on our results to a first-order approximation by considering a bidisperse system of colloids in our MC simulations. Colloids were initialized at their standard lattice positions ( g =0.12) with σ c / σ m =9.50; however, in each instance half of them were chosen at random and their diameters were decreased by 10%. Simulations were repeated 30 times to account for variations in these choices and to ensure statistical accuracy. We define polydispersity, δ , in the conventional fashion as the ratio of the standard deviation to the mean of the diameters, which yields ~5.3% for this system. Simulation model A In the case of colloids and linear polymers, we used a nearly hard-sphere potential for the colloids and monomer beads, which is amenable to simulation using traditional MD, for both our MD and MC simulations. All particles interact through a cut and translated Lennard–Jones potential: where Δ=( σ i + σ j )/2−1 and σ i refers to the diameter of the particle, cut off at r cut =Δ+2 1/6 so as to be purely repulsive. This is better known as the WCA potential [44] . Polymers are represented by a freely jointed bead-spring model where beads (Kuhn segments) are spheres with diameter σ m =1, connected by finitely extensible non-linear elastic bonds: . Following the Kremer–Grest model, we set k =30 and r 0 =1.5, which minimizes bond crossing [45] . Colloids are represented as single spheres with a diameter σ c =6.45 σ m , unless otherwise stated, which is large enough to avoid Kuhn-segment-level depletion effects and allow the beads to pass through trigonal voids created by tangent triplets of colloids [46] . Simulation model B When calculating using MC in the case of the tetramers, both beads and colloids were modelled as purely hard spheres to accelerate the calculations. Changing between WCA and hard-sphere potentials did not change our results qualitatively (and only minimally quantitatively) in the case of linear chains, so we do not expect any differences to be significant here either: where σ ij =( σ i + σ j )/2. Bonds are described as square wells according to where r m , ij denotes r end or r mid between beads i and j . Again, nearest-neighbour colloids in the crystal were placed with an additional gap of 0.12 σ m between them to be more representative of the WCA potentials used in the MD, and σ c =6.45σ m . Terminal beads had a diameter of 1.75 σ m while the interior beads had a diameter of σ m =1.0 ( cf. Fig. 4 ). These potentials were emulated in MD by replacing equation (9) with equation (8), and equation (10) with a harmonic potential: The equilibrium length for a bond is given by r 0, ij =1.05 r m , ij , and the potential strength, k ij , was set such that U bond, ij ( r m , ij ) = U bond, ij (1.1 r m , ij )=10 k B T . Simulation model C We tested other variations of pair potentials to rule out their significance. By increasing the size of the large terminal beads ( cf . Fig. 4 ) and shortening the bonds (relative to Model B) we found that kinetic barriers to nucleation and annealing were significantly reduced. In this model, terminal beads had a diameter of 2.2 σ m , while internal ones were set to σ m =1.0. Using our MC simulations we found that for tetramers with ( r mid , r end )=(1.2, 3.2) in a crystal with σ c =6.45 σ m , g =0.12 σ m , , which suggests a relatively strong preference for the FCC. All particles interacted through a hard-sphere potential ( cf . equation (9)), but the bonds were slightly shortened: where r m , ij denotes r end or r mid between beads i and j , and δ m =0.2 for r end and 0.1 for r mid . The MD counterparts for these MC simulations replaced equation (9) with equation (8) and their bonding potential, equation (12), with the harmonic potential of equation (11). Again, the bond strength was set such that U bond, ij ( r m , ij )= U bond, ij ( r m , ij + δ m )=10 k B T , and r 0, ij = r m , ij + δ m /2. How to cite this article: Mahynski, N. A. et al . Stabilizing colloidal crystals by leveraging void distributions. Nat. Commun. 5:4472 doi: 10.1038/ncomms5472 (2014).